Interstitial modification of palladium nanoparticles with boron atoms as a green catalyst for selective hydrogenation Lindlar catalysts comprising of palladium/calcium carbonate modified with lead acetate and quinoline are widely employed industrially for the partial hydrogenation of alkynes. However, their use is restricted, particularly for food, cosmetic and drug manufacture, due to the extremely toxic nature of lead, and the risk of its leaching from catalyst surface. In addition, the catalysts also exhibit poor selectivities in a number of cases. Here we report that a non-surface modification of palladium gives rise to the formation of an ultra-selective nanocatalyst. Boron atoms are found to take residence in palladium interstitial lattice sites with good chemical and thermal stability. This is favoured due to a strong host–guest electronic interaction when supported palladium nanoparticles are treated with a borane tetrahydrofuran solution. The adsorptive properties of palladium are modified by the subsurface boron atoms and display ultra-selectivity in a number of challenging alkyne hydrogenation reactions, which outclass the performance of Lindlar catalysts. Catalytic partial hydrogenation of alkynes to alkenes is a key transformation in industrial organic synthesis [1] , [2] . It is established that a solid catalyst containing palladium (Pd) in the presence of hydrogen is the most preferable choice over stoichiometric chemical reagents and homogeneous catalysts in terms of green chemistry and reusability of the catalysts. However, the surface of unmodified supported Pd metal is highly unselective, which will lead to over-hydrogenation to undesired alkanes. Traditional approaches used to tune the surface and hence the chemical reactivity of Pd include: incorporating additives, modifying support materials or alloying with other metal atoms (and also core-shell) to Pd nanoparticles. As a result, Lindlar catalysts were developed with Pb and quinoline additives to modify the Pd sites and hinder the formation of Pd hydride in the proximity of the catalyst surface [3] . Lindlar catalysts have been demonstrated to be versatile and effective and remain to be most frequently used despite their discovery over 60 years ago. However, handling toxic Pb(OAc) 2 during catalyst preparation, leaching of surface doped Pb element in the presence of substrates or products with multi-functional groups (such as drug candidates or biomass molecules), poor selectivity and limited catalyst robustness begin to restrict them from wider and new applications. In addition, the hydrogenation of monosubstituted alkynes to corresponding alkenes for the synthesis of synthons of functional polymers and total syntheses of complex molecules over Lindlar catalysts are still difficult and challenging [1] , [2] , [3] , [4] . On the other hand, much less attention is paid to modifying Pd metal using light element atoms (defined here as being elements up to the third row elements) by placing them into the subsurface interstitial lattice sites within the metal lattice structure. The changes in lattice parameter and charge transfer between the host–guest may also alter the band structure, hence catalytic properties of the supported Pd metal [5] , [6] , [7] , [8] , [9] , [10] . It is therefore interesting to develop new Pd nanocatalysts modified with interstitial atoms as a greener alternative to Lindlar catalysts for selective hydrogenation reactions. There have been few previous reports on Pd systems with interstitial atoms. By treating hydrogen gas over clean Pd at room temperature, it is known that hydrogen atoms can rapidly move into the Pd interstices due to it possessing the smallest atomic size, fast diffusion and strong chemisorption to form a Pd-β-hydride phase. Teschner et al. [5] have recently shown that interstitial C ( int C) produced in situ from adsorbed carbonaceous species at elevated temperature can be used to drastically alter the gas phase hydrogenation of alkynes. Subsurface O in Pd at high temperatures has also been demonstrated to be the kinetically active surface for CO oxidation in the high temperature regime [6] , [7] and the selective epoxidation of ethylene over silver catalysts is also thought to involve the subsurface oxygen atoms [8] . Apart from the β-hydride, it was not possible to experimentally isolate these interstitial occupied materials that were produced in situ , let alone of control and tune their content: The major technical difficulty to isolation being that these materials only exist under transient conditions in a small quantity at elevated temperatures and under an atmosphere of reactive gas. It is important to note that the infiltration of light atoms into the close packed metal lattice, though they may fit into the interstitial holes, is usually a highly activated process that requires extreme conditions that could cause sintering of high surface metal nanoparticles. To overcome the sintering problem we have synthesized a Pd- int C nanocatalyst from glucose pyrolysis where the formed carbonaceous layer can rapidly encapsulate individual Pd nanoparticles for the interstice filling during the heat treatment process [9] , [10] . However, this approach requires a complex procedure to remove the surface carbon for subsequent catalytic applications, which can also reduce the interstitial carbon content. The interstitial carbon atom in the Pd lattice is unstable, which limits its potential applications in catalysis. It is thus highly desirable to develop supported Pd catalysts modified with other interstitial atoms that are both formed under ambient conditions and are stable under mild catalytic testing conditions. The relative atomic size, the nature of chemical species, as well as the enthalpy (electronic stabilization) and entropy of surface adsorption versus lattice entrapment are all expected to be important factors. We have been interested in the synthesis of interstitial boron ( int B) to modify the metal electronic structure, and consequent catalytic activity of Pd nanocatalysts. It is intriguing to note that limited volumes of literature exist on studying the effects of subsurface boron, with research being predominately focused on the study of high temperature ordered Pd x B y alloys [11] , [12] , [13] , [14] , [15] , [16] . Although several routes to prepare interstitial B modified Pd (Pd- int B) materials have been documented [17] , [18] , [19] , [20] , none of the above have achieved a method that incorporates the criteria of low temperature synthesis, high degree of doping with int B and also importantly use a low toxicity B source equivalent, which are essential in modern catalysis synthesis. There have been some computational simulations for int B on other metal lattices and related catalysis studies, but versatile synthesis method, detailed material characterization, stability evaluation and more importantly the direct structure–activity relationship with important catalytic applications are still lacking. Here, we explore the scope of interstitial chemistry by using borane tetrahydrofuran (BH 3 .THF) as a B source for the synthesis of a Pd- int B nanocatalyst and compare this with Lindlar catalysts within a number of industrially relevant, challenging partial hydrogenation reactions. A highly doped Pd- int B phase (up to 20% of atomic B) can be synthesized at low temperature, in steep contrast compared with the traditional high temperature process for bulk material synthesis [21] . It is demonstrated that the new supported and stable Pd- int B/C nanocatalyst displays ultra-selectivity for alkyne partial hydrogenations to cis -alkenes in both the liquid and gas phase without inducing hydrogenolysis for unnecessary bond cleavage, isomerization and double bond shift that commonly occur on conventional Lindlar catalyst surfaces within delicate fine chemical or pharmaceutical applications. The dramatic enhancement in selectivity for the chemical transformations over Pd is attributed to the presence of int B. Synthesis and characterization and materials stability We began by exploring the addition of BH 3 .THF to a pre-formed sample of Pd/C ( Fig. 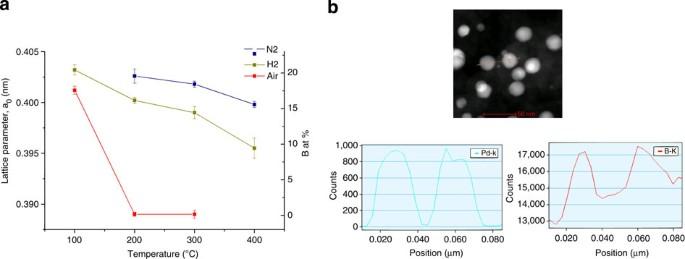Figure 1: Boron atoms incorporated into the Pd subsurface. (a) Lattice parameter, a0, measured using the average of all observablefccPd peaks from XRD (derived from lab-based X-ray diffractometer) normalized against the Al peaks from the sample cell. The error bar in lattice parameter at each temperature represents experimental error based on 3–5 repeated measurements. (b) A detailed EDX line scan of two Pd containing particles from fresh Pd(B)/C sample and corresponding X-rays counts of Pd(K) and B(K). It can be clearly seen that the B signals mirror to those of Pd showing that the signals are arisen from the Pd(B) particles (the B signal is higher than background suggesting that the support takes up B species, (refer to XPS inSupplementary Figs 1,2)). Scale bar, 50 nm. 1a , Supplementary Figs 3a,4,5 , Supplementary Table 1 , see Supplementary Notes and Supplementary Methods ). A high concentration of BH 3 .THF (25 eq. mol B to mol Pd) was used to ensure maximum B incorporation. It was interesting to see that the B doped Pd samples were significantly different compared with their non-doped counterparts from the powder X-ray diffraction (PXRD) patterns ( Supplementary Fig. 4 ). The difference was characterized by a definitive shift in XRD peaks to lower 2 θ . Similarly, lattice expansion was also obtained by doping B to CaCO 3 supported Pd, which showed that the nature of support did not seem to interfere the B incorporation ( Supplementary Fig. 6 ). But the acidity and polarity of the support could affect hydrogenation in liquid phase so inert carbon support was mainly the focus in this work. Futher XRD characterziation using synchroton radiation at the Diamond Radiation Source, UK with the application of profile refinement clearly indicated the same unit cell lattice of face-centred cubic structure (Fm3m) but with an increase in lattice parameters. This effect is indicative of B interstitial occupation leading to a clearly observed expansion of the Pd metal lattice at room temperature. 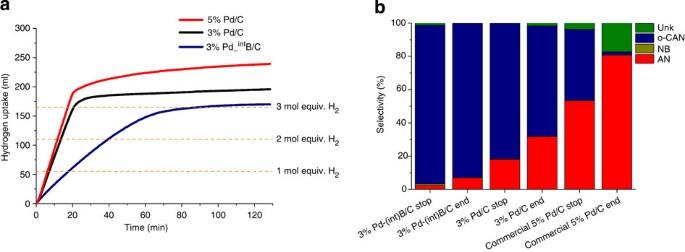Figure 2: Catalytic results of the hydrogenation ofo-CNB reaction. (a) H2uptake curves for hydrogenation ofo-CNB on: (i) commercial 5% Pd/C (red); (ii) non-modified 3% Pd/C (black); (iii) 3% Pd-intB/C (blue). Conditions: 2.46 mmol octane ando-CNB, 3.80 μmol catalysts, octane as internal standard, EtOH, 3 bar H2, 50 °C, 1,200 r.p.m., HEL ChemSCAN II Reactor. (b) GC results in the hydrogenation ofo-CNB. Stop: sample collected before rate change in the H2uptake (at 190, 170 and 155 ml H2uptake for commercial 5% Pd/C, non-modified 3% Pd/C and 3% Pd-intB/C, respectively). End: sample collected at the end of H2uptake. All samples were at 100% conversion ofo-CNB; H2uptake value of ~65 ml for 1 mol equiv.o-CNB. An unmodified Pd phase could no longer be observed when a further heat treatment at 200 °C in N 2 was used ( Supplementary Table 2 ). Additionally, EDX line scans of PdB particles under our analytical transmission electron microscope ( Fig. 1b ) clearly show the higher content B signal associated with Pd signal of selected particles from the background. This suggests that B is taken up by the Pd nanoparticle. 11 B ssNMR also indicated the presence of both boron species on surface as well as in the interstitial sites of Pd after the BH 3 .THF treatment ( Supplementary Fig. 7 ). Solid solutions of boron atoms in the interstitial sites of Pd fcc lattice with a range of composition and structure prepared by the extremely high temperature preparation method that utilizes excess arc melted B atoms to infiltrate into Pd foils have been extensively studied [17] . We have estimated the occupancy of interstitial sites from the lattice expansion to be ca. 20% ( Supplementary Equation 1 and Supplementary Table 1 ), which is comparable to the saturated value produced from the reported high temperature method [17] . It should also be noted that the intrinsic Pd fcc phase was retained with no ordered alloys observed at room temperature. We attribute the efficient low temperature process for the production of interstitial B atoms from BH 3 .THF in contact with the supported Pd nanoparticle surface partly to an entropic contribution. The adsorbed B atoms are formed initially on the Pd surface with the subsequent evolution of H 2 gas from the precursor. A strong driving force to move the surface B atoms deep into the Pd lattice is therefore expected in this case. In contrast to this low temperature process, only ~15% site occupancy of int C was achieved by our Pd nanoparticles encapsulated by glucose derived carbonaceous coating at high temperature regardless of the particle size, where the carbon saturation was reached [13] . It is interesting to note that comparison of the atomic radii between the light elements (H, B, C, N and O), B is the largest atom and yet the formation of Pd- int B with atomic fraction is remarkably higher than C and causing larger lattice expansion (~3.6% versus ~2.3% in lattice parameter) and can be carried out using such a mild temperature treatment. Figure 1: Boron atoms incorporated into the Pd subsurface. ( a ) Lattice parameter, a 0 , measured using the average of all observable fcc Pd peaks from XRD (derived from lab-based X-ray diffractometer) normalized against the Al peaks from the sample cell. The error bar in lattice parameter at each temperature represents experimental error based on 3–5 repeated measurements. ( b ) A detailed EDX line scan of two Pd containing particles from fresh Pd(B)/C sample and corresponding X-rays counts of Pd(K) and B(K). It can be clearly seen that the B signals mirror to those of Pd showing that the signals are arisen from the Pd(B) particles (the B signal is higher than background suggesting that the support takes up B species, (refer to XPS in Supplementary Figs 1,2 )). Scale bar, 50 nm. Full size image In the late 1930s, Hägg and coworkers predicted the maximum size of interstitial atoms that could be accommodated in a lattice, with the assumptions that the interstitial atoms are totally inert with no interaction with host atoms and do not disrupt lattice packing as a truly solid solution. Theoretically, no solid solution should ever be formed between Pd and B, according to the Hägg’s criterion, the critical atomic radius ratio between the light element ( r i ) and the metal ( r m ) is satisfied only if the atomic radius ratio ( r i /r m ) is <0.59 ( r B /r Pd =0.67) [17] . Apparently, the hard sphere model is inconsistent with the observed volume–interstitial content relationship for the interstitial solid solution Pd- int B: a significant, negative deviation from the hard sphere model prediction (volume contraction) occurs. It was concluded that the chemical (electronic) interaction appears to govern the interstitial solid solution formation rather than the elastic interaction as characterized by the Hägg atomic radius ratio or the volume size factor. Furthermore, it is energetically disfavoured to expand the metal lattice and therefore apart from the entropic contribution, extra energy stabilization must be needed for the migration of such light atoms from metal surface to interstitial sites (further discussion on Hagg’s and King’s size criteria is in Supplementary Discussion ). It is believed that this extra stabilization must come from a direct electronic interaction with the host lattice atoms, the mixing of the B s-p orbitals with Pd d -orbitals (DFT calculations shown later). Consequently, we investigated the stability of the new Pd- int B phase by determining the amounts of int B retained in Pd after exposure to a series of reactive gases, as measured by their shifts in lattice parameter ( Fig. 1a and Supplementary Figs 4,5,8–10 and calculation method used). Interestingly, significant differences were observed when the Pd- int B/C was heat treated under different gaseous atmospheres. It can be seen that no metallic Pd peak (with an unmodified lattice parameter) was evident under N 2 at 200 °C, where maximum boron incorporation (lattice expansion of 3.6%) was maintained. When Pd- int B/C was treated in air, a clear loss of boron was observed at their analogous temperatures. The content of Int B was attenuated under oxidising conditions but there was only marginal loss of boron in H 2 atmosphere at above 200 °C (see temperature programmed reduction with mass spectrometry ( Supplementary Fig. 11 ). Nevertheless, there was no loss in B under a flowing stream of hydrogen over the temperature range of 100–150 °C at prolonged time of testing, which suggests Pd- int B/C catalyst is stable to be used under the conditions for most selective chemical transformations of fine and speciality chemicals, as we targeted it for. On comparing these values with the class of Pd- int C catalysts studied [22] , [23] , it is apparent that the Pd- int B nanocatalysts exhibit much higher thermal stability under a reducing atmosphere than the Pd- int C catalyst, as all the int C are readily converted to CH 4 at 150 °C under a reducing atmosphere. Therefore, the higher apparent thermal stability of Pd- int B and higher degree of interstitial filling at milder conditions could be ascribed to a corresponding higher degree of orbital interaction, leading to its increased stability compared with Pd- int C. It is apparent that Pd- int B/C can be handled in air at or below 100 °C without phase segregation; however, at more elevated temperatures significant decomposition of the Pd- int B phase was observed. Heat treating the catalyst in air at ≥200 °C resulted in ejection of int B with simultaneously reformation of metallic Pd, boron migration from subsurface is likely to have been induced through oxidation of boron atoms with adsorbed oxygen that remained on the surface of Pd (see temperature programmed oxidation with mass spectrometry, Supplementary Figs 12,13 ). Chemisorbed oxygen has a propensity to induce phase segregation, as there is a stronger binding affinity of B for O than Pd [24] . As a result, one should be cautious of examining this type of catalysts for reactions under different gas atmospheres at unsustainable high temperatures. 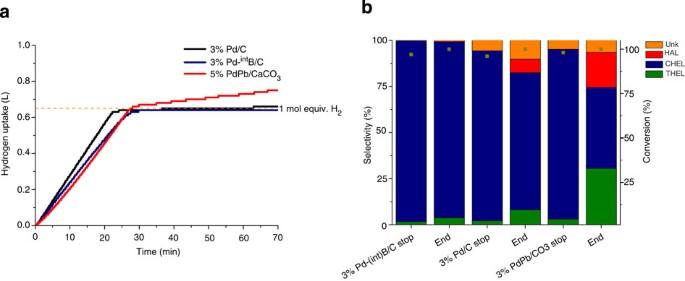Figure 3: Catalytic results of the hydrogenation of 3-hexyn-1-ol reaction. (a) Hydrogen uptake curves in the hydrogenation of 3-hexyn-1-ol for: (i) non-modified 3% Pd/C (black); (ii) Pd-intB/C (blue); (iii) Lindlar’s 5% PdPb/CaCO3(red). Conditions: 30 mmol 1,4-dioxane and 3-hexyn-1-ol, 2.80 μmol catalyst in EtOH, 3 bar H2, 30 °C, 400 r.p.m., Parr autoclave. H2uptake value of ~650 ml for 1 mol equiv. to alkyne. (b) GC results for the stereoselective hydrogenation of 3-hexyn-1-ol. Stop: sample collected before the change in hydrogen uptake. End: sample collected at the end of hydrogen uptake. THEL, trans-hexen1-ol; CHEL, cis-hexen-1-ol; HAL, 1-hexanol. Yellow dot represents percent of conversion. Extended X-ray absorption fine structure (EXAFS) fitted parameters are shown in Supplementary Equation 1,3 and Supplementary Table 3 . It can be seen from the fitted data that addition of B clearly leads to an expansion of the average Pd–Pd distance, as evidenced by the reduced amplitudes from the EXAFS oscillations ( Supplementary Fig. 14 ). The degree of lattice expansion suggests that B is indeed occupied in the octahedral holes of Pd, this fact is consistent to the PXRD data [25] . The structure of Pd remained in the fcc structure in agreement with the PXRD. The interatomic distance increased upon addition of B in Pd. This result was in line with the previous study where Pd foil was homogenized with atomic B followed by rapid quenching to form Pd-B [25] . The coordination number apparently decreased on addition of B, albeit the lower value for Pd/C falls within the upper value for Pd- int B/C. The amount of B in the sample determined from the lattice parameter was estimated at 11.3% in contrast with 20% B estimated by PXRD, which could reflect the difference in sensitivity to Pd sizes and their variations in B loadings by the two measurements. It is noted that the fitting of EXAFS data could be marginally improved by adding an extra-shell of B (Pd–B interaction) but this analysis was not included with taking experimental errors into consideration due to B being an extremely poor X-ray absorption (despite the high B/Pd signals shown in the EDX line scans of the Pd(B) particles ( Supplementary Fig. 15 ). Catalytic performance It is important to establish whether these new Pd- int B nanoparticles supported on activated carbon or calcium carbonate with electronically-modified Pd by the subsurface B atoms can be of any significance for selective hydrogenation transformations under mild conditions. Selective partial hydrogenation of fine and speciality chemicals in the liquid phase was chosen as these present significant challenges for ultra-selectivity (delicate molecules may easily undergo side reactions that need to be eliminated). First, partial hydrogenation of chloro-nitrobenzene (CNB) to chloroaniline (CAN) without hydrodechlorination (to avoid hydrogenolysis of the facile aryl-Cl bond is a key challenge) was investigated. This hydrogenation represents an important class of chemical transformation towards the manufacture of dyes, pharmaceuticals, polymers, herbicides and pesticides [26] . Most studies in the literature have focused on using Pt-based catalysts to achieve high CNB hydrogenation while at the same time maintaining low rates of hydrodechlorination [27] , [28] , [29] . Meanwhile, conventional Pd based catalysts generally offer significantly lower selectivity due to aryl-chloride bond cleavage [30] , [31] , [32] . Furthermore, the poor activity and severe leaching of Pb to form PbCl 2 render Lindlar catalysts totally unsuitable for this application [1] , [32] . However, there is a strong economic advantage to use Pd instead of Pt in this application, due to the lower costs of the former. Recently, studies have been devoted on maximizing CAN selectivity either by, to name but a few, alloying [7] , [33] , incorporating additives [34] or using different metal supports to Pd [26] . Therefore, the versatility of this new class of catalyst was investigated for the partial hydrogenation of o -CNB to o -CAN ( Supplementary Fig. 16 ) as compared with a commercial 5% Pd/C, a non-modified 3% Pd/C and a corresponding 3% Pd- int B/C catalyst. Figure 2a shows the H 2 uptake curves for those catalysts tested under industrially applicable conditions. A higher initial activity was observed for the commercial 5% Pd/C and is attributed to the smaller particle sizes (~5 nm) compared with the non-modified 3% Pd/C catalysts. 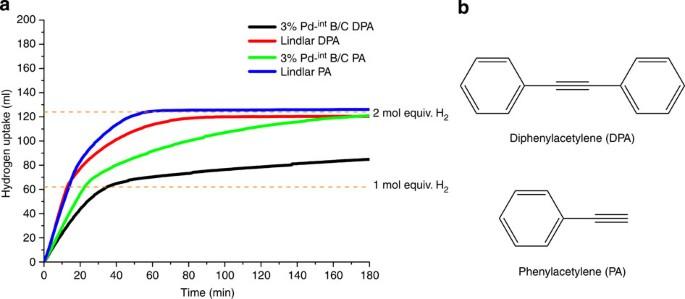Figure 4: Catalytic results of the hydrogenation reactions of various non-polar substituted alkyne. (a) Hydrogen uptake curves in the hydrogenation of (i) Diphenylacetylene (DPA) over Pd-intB/C catalyst (black); (ii) DPA over Lindlar’s catalyst (red); (iii) Phenylacetylene (PA) over Pd-intB/C catalyst (green); (iv) PA over Lindlar’s catalyst (blue). Conditions: 2.50 mmol alkyne, 2.50 μmol catalyst, EtOH, 3 bar H2, 30 °C, 1,200 r.p.m. H2uptake value of ~62 ml for 1 mole equiv. to alkyne. (b) Structure of substrate molecule (top: DPA, bottom: PA). The initial activity for 3% Pd- int B/C was lower than that of the unmodified catalyst, indicating a partial loss of surface area after B addition ( Supplementary Table 4 ). However, the large difference in the initial activity between Pd/C and Pd- int B/C could not be entirely due to the loss in metal sites but the modified surface electronic structure by B incorporation. 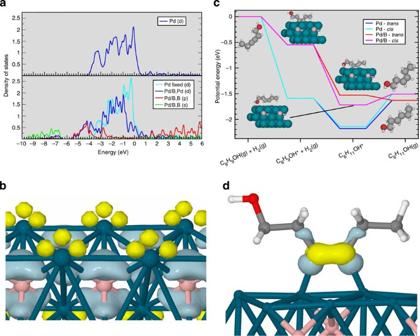Figure 5: Density functional theory study of Pd-intB system. (a) Density of states diagram of pure Pd (upper part of panel);d-states of Pd with frozen displacement (cyan);d-states of Pd withintB (blue);p-states of B in Pd (red); s-states of B in Pd (green; lower part of panel); (b) an electron density difference isosurface plot showing local electron richer (light blue) and poorer regions (yellow) of Pd atoms (blue) withintB atoms (pink) due to states-mixing (−'ve/+'ve density units=±0.05 electron per angstrom cube); (c) potential energy profile of 3-hexyn-1-ol adsorbed on a (2x4)-Pd(111) unit cells of 3-atomic layers on clean Pd and Pd-intB and (d) isosurface of isolated molecular Highest Occupied Molecular Orbital/Lowest Unoccupied Molecular Orbital (HOMO/LUMO) (blue/yellow, respectively) superimposed on the adsorbate/surface structure (units=0.3 electron per angstrom cube). Figure 2b and Supplementary Table 5 shows the gas chromatography analysis at the rate change in H 2 uptake and at the end of the reaction. Notice that the commercial 5% Pd/C sample gave only 42.8% selectivity towards o -CAN. The catalyst appeared to yield excessive hydrodechlorination as evidenced by the higher selectivities towards aniline (31.7%) and unknown products (1.8% unkown) being isolated as the main by-products. Analysis at the end of the reaction led to almost no selectivity towards the partial hydrogenated product o -CAN (1.8%), which was accompanied by observation of higher boiling point diazo products due to excessive adsorption of intermediate(s) and catalysis on surface. In contrast, a higher selectivity to o -CAN (81.3%) was obtained over 3% Pd/C with a larger average Pd particle size (13 nm). Upon comparing the 3% Pd- int B/C with non-modified 3% Pd/C of a similar particle size but with the B inclusion ( Supplementary Table 5 ), it was clear that Pd- int B gave a much enhanced selectivity to o -CAN of 95.4%, the difference in their selectivity became larger towards the end of the reaction (an increase to 27%). In addition, no formation of higher boiling by-products was observed for the Pd- int B/C. This result clearly demonstrates that the Pd- int B gives the ability to suppress the delicate hydrodechlorination pathway despite the failure of using Lindlar catalysts, which may be used as an alternative for Pt based catalysts in the chemoselective hydrogenation of o -CNB to o -CAN. Figure 2: Catalytic results of the hydrogenation of o -CNB reaction. ( a ) H 2 uptake curves for hydrogenation of o -CNB on: (i) commercial 5% Pd/C (red); (ii) non-modified 3% Pd/C (black); (iii) 3% Pd- int B/C (blue). Conditions: 2.46 mmol octane and o -CNB, 3.80 μmol catalysts, octane as internal standard, EtOH, 3 bar H 2 , 50 °C, 1,200 r.p.m., HEL ChemSCAN II Reactor. ( b ) GC results in the hydrogenation of o -CNB. Stop: sample collected before rate change in the H 2 uptake (at 190, 170 and 155 ml H 2 uptake for commercial 5% Pd/C, non-modified 3% Pd/C and 3% Pd- int B/C, respectively). End: sample collected at the end of H 2 uptake. All samples were at 100% conversion of o -CNB; H 2 uptake value of ~65 ml for 1 mol equiv. o -CNB. Full size image The stereoselective partial hydrogenation of 3-hexyn-1-ol to the corresponding cis -hexen-1-ol (CHEL) was also chosen for the study as this typical reaction has significant importance in the fragrance industry towards the manufacturing of leaf fragrance alcohol ( Supplementary Fig. 17 and Supplementary Table 6 ) [35] . Even trace levels of undesirable over-hydrogenated products and other isomers would greatly alter the aroma of the mixture. The reaction progress was monitored by measuring the H 2 uptake against time under the same conditions ( Fig. 3a ). It was found that all catalysts gave good activity, reaching the semi-hydrogenation point after 20 min. An induction period was observed in the initial stages of H 2 uptake for the Lindlar catalyst, as characterized by the curve having a slight parabolic shape that suggests that the catalyst was initially in the oxidized state [36] . Aliquots were taken at points where the reaction reached the semi-hydrogenation theoretical uptake point (1 mol equiv. of H 2 uptake with respect to alkyne) and also at the end of the reaction, for analysis by gas chromatography ( Fig. 3b ). When comparing the catalysts, it was found that the 3% Pd- int B/C was again the most selective towards CHEL (98%) as characterized by the very high cis / trans ratio at the half H 2 uptake point (53.5). It is interesting that virtually no over-hydrogenation products were observed for Pd- int B/C as no hexanol (HAL) was detected. The selectivity towards CHEL and cis / trans ratio are apparently higher than that of Pd- int C catalysts we reported earlier (91.9% CHEL, cis / trans ratio of 10.8) under the comparable conditions [9] , [10] suggesting that int B is more effective than int C in subsurface modification of Pd for this reaction. On the other hand, both 3% Pd/C and surface poisoned Lindlar catalyst suffered from the significant over-hydrogenation to HAL as well as a rapid isomerization to trans -hexen-1-ol. The adsorption strength of alkyne on metal surface is generally much higher than corresponding alkene molecules, thus modification by interstitial atoms or surface dopings to reduce the adsorptive ability of Pd are known to be beneficial to give higher selectivity towards alkenes ( cis and trans ) at high conversion (the metal surface is primarily covered with alkyne molecules). But after the conversion of alkyne, the fine tuning of metal surface is very important to reduce the further conversion of desirable cis alkene by weakening its absorption (reduction in isomerization reactions to trans or double bond shift of the adsorbed molecule). It is clear from our results that the use of the longer contact time in hydrogen in the batch reactor after the half hydrogen uptake allowed for further isomerizations to take place for all the catalysts but the high cis / trans ratio at the end of experiment in the case of Pd- int B/C ( cis / trans ratio=25.4) clearly suggests that the extent of isomerization over this catalyst is not prominent. Comparatively, at the end of reaction, the Lindlar catalyst gave 43.9% CHEL with 30.6% towards HAL with cis / trans ratio of 1.4. Thus, the Pd- int B/C gave much reduced isomerization rate compared with the non-modified 3% Pd/C with the Lindlar catalyst, the highest of all three catalysts. An increase in the rates of over-hydrogenation and isomerization for Pd/C and Lindlar catalyst is attributed to the uncompromized stronger adsorption of the partial hydrogenated product on the catalyst surfaces due to characteristic d -band positions (see DFT calculations) and partly to the hydrophilic nature of support with higher affinity for hydrophilic substrate. Whereas the Pd- int B/C (non-hydrophilic) with modified electronic band structure by the boron atoms greatly reduced the residence time for substrate adsorption (weaker adsorption) and hence importantly much lower isomerization rates. Figure 3: Catalytic results of the hydrogenation of 3-hexyn-1-ol reaction. ( a ) Hydrogen uptake curves in the hydrogenation of 3-hexyn-1-ol for: (i) non-modified 3% Pd/C (black); (ii) Pd- int B/C (blue); (iii) Lindlar’s 5% PdPb/CaCO 3 (red). Conditions: 30 mmol 1,4-dioxane and 3-hexyn-1-ol, 2.80 μmol catalyst in EtOH, 3 bar H 2 , 30 °C, 400 r.p.m., Parr autoclave. H 2 uptake value of ~650 ml for 1 mol equiv. to alkyne. ( b ) GC results for the stereoselective hydrogenation of 3-hexyn-1-ol. Stop: sample collected before the change in hydrogen uptake. End: sample collected at the end of hydrogen uptake. THEL, trans-hexen1-ol; CHEL, cis-hexen-1-ol; HAL, 1-hexanol. Yellow dot represents percent of conversion. Full size image Hydrogenation of non-polar substituted alkyne (for example, diphenylacetylene (DPA)) was also examined in ethanol over both Lindlar catalyst and 3% Pd- int B/C ( Fig. 4 ). The reaction progress was again followed by monitoring the H 2 uptake ( Fig. 4 , conditions: HEL ChemSCAN, three bar H 2 (excess H 2 ) 30 °C, 2.50 μmol catalyst, 0.5 M alkyne in 5 ml EtOH, 1,200 r.p.m., 1,000:1 substrate to metal ratio). The rate difference between H 2 uptakes before/after 1 mol equiv. of H 2 consumption (~62 ml of H 2 in this case) gave an indication of semi-hydrogenation selectivity to the alkene, as aforementioned (only the semi- and fully-hydrogenated products were detected). The Lindlar catalyst exhibited almost the same initial activities and selectivities for this alkyne hydrogenation as 3% Pd- int B/C at the inflection point of 65 ml where 1 mol equiv. H 2 consumption was reached (89.7% DPA conversion, 94.3% selectivity to stilbene (alkene products with cis/trans=32.7) and 5.7% selectivity to diphenylethane (alkane) for Lindlar catalyst). However, a much poorer hydrogenation selectivity was observed towards stilbene at longer time as the catalyst continued to hydrogenate towards the saturated alkane beyond the semi-hydrogenation point until reaching the total consumption of 2 mol equiv. of H 2 (~124 ml of H 2 ) with virtually 100% yield to diphenylethane. The over-hydrogenation on corresponding terminal alkyne, the phenylacetylene (PA) was even more prominent as there was no inflection near the equivalent semi-hydrogenation region to quench the reaction to alkene (styrene) in the hydrogenation curve ( Fig. 4 ) but the hydrogenation rapidly proceeded to completion, giving 100% yield to alkane product (ethyl-benzene). This is not surprising as non-polar mono-substituted alkynes, as previously stated, are in general significantly more difficult to hydrogenate to unsaturated alkenes due to their smaller difference in adsorption strength on the metal surface [4] . It is noted that unsatisfactory results were obtained with the use of Lindlar catalyst over such non-polar alkynes hydrogenation in alcoholic solvents [1] . An elaborate set-up to restrict access of hydrogen gas and to monitor the reaction progress is commonly required to reduce the excessive over-reduction to alkanes. In addition, delicate adjustment of surface concentration of lead acetate, depending on nature of substrate, to avoid over poisoning the Pd/CaCO 3 catalyst is needed. It is often observed that hydrogenations over Lindlar catalysts proceeded not at all or only very slowly [1] . Figure 4: Catalytic results of the hydrogenation reactions of various non-polar substituted alkyne. ( a ) Hydrogen uptake curves in the hydrogenation of (i) Diphenylacetylene (DPA) over Pd- int B/C catalyst (black); (ii) DPA over Lindlar’s catalyst (red); (iii) Phenylacetylene (PA) over Pd- int B/C catalyst (green); (iv) PA over Lindlar’s catalyst (blue). Conditions: 2.50 mmol alkyne, 2.50 μmol catalyst, EtOH, 3 bar H 2 , 30 °C, 1,200 r.p.m. H 2 uptake value of ~62 ml for 1 mole equiv. to alkyne. ( b ) Structure of substrate molecule (top: DPA, bottom: PA). Full size image On the other hand, for 3% Pd- int B/C catalyst with intrinsic interstitial B modification, at the equivalent 1 mol of hydrogen uptake there was slightly higher degree of conversion of DPA to stilbene with higher cis / trans ratio (91.4% DPA conversion, 93.8% selectivity to stilbene ( cis / trans =35.1) and 6.1% selectivity to diphenylethane). Clearly in accordance with Fig. 4 , the rate of over-hydrogenation of the DPA molecule beyond 1 mol hydrogen equivalent was very slow, giving similar stilbene selectivity even in excess of hydrogen atmosphere at prolonged time. In addition, the over-hydrogenation of the more challenge terminal PA alkene over the 3% Pd- int B/C catalyst was still continued in excess hydrogen (at 1 mol H 2 equivalent, 100% PA conversion, 92.9% selectivity to styrene, 7.1% selectivity to ethyl-benzene until reaching 2 mol H 2 equivalent with 100% yield to ethyl-benzene) but at a much lower rate as seen from the slower H 2 uptake curve, which can be alleviated by limiting the access of hydrogen or/and time due to a clear difference in the rates for the first and second hydrogenations. By using CaCO 3 as a support, though it is more polar than that of carbon support, a similar trend of 5% Pd- int B/CaCO 3 was also obtained compared with 5% Pd/CaCO 3 for the slower rate for over-hydrogenation of alkene in the hydrogenation of DPA or PA ( Supplementary Fig. 18 and Supplementary Table 7 ). Again, the hydrogenation of DPA molecule beyond 1 mol hydrogen equivalent was very slow, giving higher stilbene selectivity and cis / trans ratio than that of the boron absent Pd sample even in excess of hydrogen atmosphere at prolonged time. These results clearly demonstrate that the boron modified catalysts despite the use of different supports indeed show a dramatic, beneficial effect of ultra-selectivity in typical partial hydrogenation reactions, even for highly challenging non-polar substrates in liquid phase. This type of catalyst did not seem to deactivate in given short testing time (within few hours) in lab scale and there was also no significant loss in B content in post-mortal catalyst analysis ( Supplementary Fig. 15 ). Surface and subsurface contributions The overall boron modification effect leading to ultraselectivity towards partial hydrogenated products may be derived from a number of contributing factors. These may include surface electronic effects, interstitial electronic effects and selective site blockage by the boron modification. Krawczyk et al. [37] studied the effect of surface B (borides and borates) in the hydrogenation of alkynes. They observed a degree of promoted alkene selectivity over alkane products by boron adspecies, which suggests that a selective surface blockage mechanism can be taken place. As a result, we have briefly studied the hydrogenation of 4-octyne ( Supplementary Equations 12–18 and Supplementary Fig. 19,20 ) over Pd- int B/C with and without interstitial boron (removal of int B selectively by 200 °C treatment in O 2 as indicated by PXRD but XPS indicated that the catalyst contained surface boron species). Remarkably, the rate ratios for the catalyst with int B removed led to a substantial decreased in selectivity ( Supplementary Table 8 ). This clearly suggests that int B has a significant role on minimizing over-hydrogenation and isomerization processes. DFT calculations As previously shown, placing boron atoms in the interstices of Pd lattice can create simultaneous electronic modification to the Pd band structure by lattice expansion and electronic interaction between intimate atoms. To appreciate their contributions we have turned to DFT calculations. Figure 5a illustrates the density of states for our clean surfaces, the top part of the panel shows the projected d -band of the surface Pd in clean Pd(111), whereas the bottom part of the panel shows the d -band of Pd in the absence of the p-block element (but frozen with the displacement induced by the p-block element), the d -band of the surface Pd in Pd/B and finally the p - and s -band of boron. This allows one to consider, firstly, the influence of expansion in the Pd lattice on the d -band, where as expected the d -band shifts up and narrows ( d -band centre/width (eV). −1.37/1.00 as compared with −1.52/1.14 (pure)). This band uplift should in principle strengthen the adsorption strength of the substrate/intermediate molecules on surface [38] , which apparently contradicts to what was observed experimentally (much weakened in adsorption). On the other hand, the influence of introducing interstitial boron appeared to facilitate an effective overlap of d - and p -bands leading to downshifts the position of d -band centre and a corresponding band broadening ( d -band centre/width (eV). −2.05/1.56 ( int B)). One would expect a similar electronic effect between boron and Pd on surface but the extensive electronic interaction of interstitial boron with parent Pd lattice is thought to be more substantial. Figure 5b clearly shows the electron enrichment of subsurface region of int B atoms indicating that it is energetically favourable to place B atom in octahedron site as a strong host–guest electronic interaction. Thus, it is believed that the overriding effect is the Pd d -band broadening and down-shifting with a good degree of state mixing from the interstitial boron atoms in sub-layers, which provide a strong stabilization to this solid solution system. The occupancy of the interstitial boron atoms can displace the H atoms (Pd hydride) at the same sites to reduce undesirable over-hydrogenation by subsurface hydrogen [39] and dramatically attenuate the adsorptivity of the metal surface to achieve ultra-selectivity in partial hydrogenation. A similar effect for electronic modification of Pd by surface Pb in Lindlar catalysts to destabilize the subsurface hydride formation has been proposed [3] . But, the conversion of 3-hexyn-1-ol to CHEL with higher selectivity over Pd- int B/C than Lindlar catalyst ( Fig. 3 ) clearly suggests the more effectiveness of subsurface B modification. Figure 5: Density functional theory study of Pd- int B system. ( a ) Density of states diagram of pure Pd (upper part of panel); d -states of Pd with frozen displacement (cyan); d -states of Pd with int B (blue); p -states of B in Pd (red); s-states of B in Pd (green; lower part of panel); ( b ) an electron density difference isosurface plot showing local electron richer (light blue) and poorer regions (yellow) of Pd atoms (blue) with int B atoms (pink) due to states-mixing (−'ve/+'ve density units=±0.05 electron per angstrom cube); ( c ) potential energy profile of 3-hexyn-1-ol adsorbed on a (2x4)-Pd(111) unit cells of 3-atomic layers on clean Pd and Pd- int B and ( d ) isosurface of isolated molecular Highest Occupied Molecular Orbital/Lowest Unoccupied Molecular Orbital (HOMO/LUMO) (blue/yellow, respectively) superimposed on the adsorbate/surface structure (units=0.3 electron per angstrom cube). Full size image We have also calculated simplified reaction profiles for the partial hydrogenation of 3-hexyn-1-ol to the corresponding cis and to trans forms in order to appreciate the high cis / trans ratio over the Pd- int B ( Fig. 5c ). In the gas phase, the total energy calculations yielded an energetic preference from the substrate hydrogenation to trans conformation by 0.14 eV than the cis product, within the realms of DFT error (±0.1 eV) that corresponds to an equilibrium constant of 225 (300 K) between trans and cis . However, if we take the substrate molecule to the surface, it will then favourably be converted to cis conformation in the energetic sequence of E ads (Pd)>E ads (Pd- int B). As the adsorptive strength of Pd- int B surface is much weaker than Pd/C (broadening and downshift of d-band, see Fig. 5b,d ), which will encourage desorption of the cis -alkene to take place (following similar arguments by Norskov and co-workers [38] for selective acetylene hydrogenation [40] ). Notice that there is a breaking degeneracy to the favouring of a cis species by 0.17 eV corresponding to an equilibrium constant of 706 (300 K), which is a sharp contrast with the noncatalysed gas phase that favours the trans form ( Supplementary Equations 4–11 ). Given the stability and similarly in calculated cis and trans energy and the existence of lower H barriers on pure Pd system (via β-hydride) as well as Lindlar catalyst (much smaller energetic preference than Pd- int B is anticipated), we would expect to see their higher degree of isomerization as observed experimentally (see Fig. 3 ). In conclusion, we demonstrate that a low temperature incorporation of boron atoms into the metal lattice of supported Pd nanoparticles is favourable due to the strong electronic interaction within the host–guest sites using BH 3 .THF as a modifying reagent. This simple chemical modification can be applied directly to existing metal supported catalysts. It is also shown for the first time that the Pd metal modified with subsurface boron atoms as a catalyst can give ultra-selectivity in selected partial hydrogenation reactions, outperforming those of Lindlar catalysts and Pd- int C in the liquid phase owing to the stronger electronic perturbation to the parent metal atoms. With regards to the growing demands for greener catalysts in partial hydrogenations and the limitations of Lindlar catalysts, the subsurface modification of Pd with boron atoms may thus find new uses in catalytic applications for fine-tuning adsorptivity/reactivity over the conventional surface methods. Synthesis of Pd/C A known amount of palladium (II) nitrate solution (15.11% Pd assay, Johnson Matthey) was dissolved in n -butanol and impregnated dropwise into a butanoic solution of Norit GSX activated carbon (Johnson Matthey) to achieve the desired theoretical metal loading. n -butanol was used as solvent because the hydrophobic properties of water may have a detrimental effect to the final metal particle size. This was stirred overnight after which the suspension was filtered and washed with copious amount of water followed by ethanol. A non orange coloured filtrate indicated anchoring of palladium onto the activated carbon support. The catalyst was dried at 80 °C in the oven overnight. Reduction of the dried catalyst was conducted in a 50:50 hydrogen to nitrogen atmosphere at a flow rate of 60 ml min −1 . The furnace was programmed using a ramp rate of 5 °C min −1 up to 500 °C and held for 1 h. The furnace was then cooled back to room temperature. Supplementary Fig. 3 shows the transmission electron microscope image of Pd/C after reduction. The average metal crystallite size was found to be 13±3 nm. Synthesis of Pd- int B/C The preparation of Pd- int B/C nanocatalysts was performed in a three-neck round bottom flask equipped with hydrogen and nitrogen switch, rubber bung and an oil bubbler. Typically, 3% Pd/C (250 mg, 0.07 mmol) was added, purged with nitrogen gas and then evacuated overnight for 20 h in vacuum at 80 °C to ensure that any residual oxygen or moisture do not prematurely oxidize the BH 3 .THF added at later time. Catalyst was then pretreated in situ at 100 °C for 1 h then cooled down to room temperature in hydrogen. 2 ml of tetrahydrofuran was added to pre-wet the catalyst followed by a dose of BH 3 .THF solution (1.8 ml, 1.76 mmol, Aldrich). The mole ratio of Pd to BH 3 .THF was 1:25. The flask was warmed to 40 °C to aid solvent evaporation before measurement. How to cite this article: Chan, C. W. A. et al. Interstitial modification of palladium nanoparticles with boron atoms as a green catalyst for selective hydrogenation. Nat. Commun. 5:5787 doi: 10.1038/ncomms6787 (2014).